Genomic footprints of activated telomere maintenance mechanisms in cancer Cancers require telomere maintenance mechanisms for unlimited replicative potential. They achieve this through TERT activation or alternative telomere lengthening associated with ATRX or DAXX loss. Here, as part of the ICGC/TCGA Pan-Cancer Analysis of Whole Genomes (PCAWG) Consortium , we dissect whole-genome sequencing data of over 2500 matched tumor-control samples from 36 different tumor types aggregated within the ICGC/TCGA Pan-Cancer Analysis of Whole Genomes (PCAWG) Consortium to characterize the genomic footprints of these mechanisms. While the telomere content of tumors with ATRX or DAXX mutations (ATRX/DAXX trunc ) is increased, tumors with TERT modifications show a moderate decrease of telomere content. One quarter of all tumor samples contain somatic integrations of telomeric sequences into non-telomeric DNA. This fraction is increased to 80% prevalence in ATRX/DAXX trunc tumors, which carry an aberrant telomere variant repeat (TVR) distribution as another genomic marker. The latter feature includes enrichment or depletion of the previously undescribed singleton TVRs TTCGGG and TTTGGG, respectively. Our systematic analysis provides new insight into the recurrent genomic alterations associated with telomere maintenance mechanisms in cancer. Telomeres are nucleoprotein complexes at the ends of chromosomes that prevent DNA degradation and genome instability [1] . The typically 10–15 kb long chromosome termini are composed of long stretches of TTAGGG (t-type) repeat arrays with an increasing number of variants toward proximal, subtelomeric regions, the most common being TGAGGG (g-type), TCAGGG (c-type), and TTGGGG (j-type) repeats [2] , [3] . Telomeres play an important role in cellular aging, as they are shortened with each cell division and finally trigger a DNA damage response resulting in senescence [4] , [5] . To avoid this permanent growth arrest, cells with unlimited proliferative potential need to extend their telomeres. In humans, telomeric DNA is synthesized by telomerase, an enzyme that is composed of the reverse transcriptase TERT and the RNA template TERC. This complex is active in the germline and stem cells, but absent in most somatic cells [6] . Telomerase is upregulated in ~85% of human cancers by different genetic aberrations, including TERT amplifications [7] , rearrangements [8] , or mutations in the TERT promoter [9] , [10] . The remaining tumors employ an alternative lengthening of telomeres (ALT) pathway, which is based on DNA recombination of telomeric sequences [11] . Details on the ALT mechanism remain elusive, but it has been associated with loss-of-function mutations in the chromatin remodeling genes ATRX (α-thalassaemia/mental retardation syndrome X-linked) and DAXX (death domain-associated protein) [12] . Telomeres of ALT cells characteristically have heterogeneous lengths and contain a range of telomere variant repeats (TVRs) [13] , [14] , [15] . Other hallmarks of ALT include ALT-associated promyelocytic leukemia nuclear bodies, abundance of extrachromosomal telomeric repeats of various forms (such as C-circles), and genome instability [11] , [16] . While normally located at the chromosome termini, telomere sequences are also found within chromosomes. As such, interstitial telomeric sequences with large blocks of telomere repeats exist in humans and other species, which probably arose from ancestral genome rearrangements or other evolutionary events [17] . Recently, also ALT-specific, targeted telomere insertions into chromosomes have been described that lead to genomic instability [18] . Another source for unexpected telomere repeat occurrence is the stabilizing function of telomeres at broken chromosomes. After a double-strand break, telomeres can be added de novo to the unprotected break sites (“telomere healing”) [19] , [20] or acquired from other chromosomal positions (“telomere capture”) [21] , [22] . The here presented study was conducted within the scope of the ICGC/TCGA Pan-Cancer Analysis of Whole Genomes (PCAWG) Consortium, which aggregated whole-genome sequencing (WGS) data from 2658 cancers across 38 tumor types generated by the ICGC and TCGA projects. This data was reanalyzed with standardized, high-accuracy pipelines to align to the human genome (reference build hs37d5), and identify germline variants and somatically acquired mutations, as described in ref. [23] . Here, we characterize the telomere landscape of 2519 tumor samples from 36 different tumor types using the WGS alignments, somatic mutation, and chromothripsis calls provided by the PCAWG Consortium [23] , [24] . Besides determining telomere content and searching for mutations associated with different telomere maintenance mechanisms (TMMs), we systematically detect 2683 somatic telomere insertions and show that different TMMs are associated with the enrichment of previously undescribed singleton TVRs. Telomere content across cohorts Due to the repetitive nature of telomere sequences, short sequencing reads from telomeres cannot be uniquely aligned to individual chromosomes. However, a mean telomere content for the tumor as a whole can be estimated from the number of reads containing telomere sequences [25] . Here, we extracted reads containing at least six telomere repeats per 100 bases, allowing the canonical telomere repeat TTAGGG and the three most common TVRs TCAGGG, TGAGGG, and TTGGGG. The telomere content was defined as the number of unaligned telomere reads normalized by sequencing coverage and GC content. Of the 2583 high-quality tumor samples available in PCAWG, we selected those from donors with a single tumor sample. From each donor, a control sample was available. In most cases this consisted of a blood sample, but could also stem from tumor-adjacent or other tissue [23] . The telomere content was determined for the remaining 2519 tumor samples and matched controls from 36 different tumor types. Several of these tumor types were not covered in a recent pan-cancer overview of telomere lengths [26] , including medulloblastoma, pilocytic astrocytoma, chronic lymphocytic leukemia, pancreatic endocrine cancers, benign bone cancer, and osteosarcoma. All relevant donor information and results used in this study are summarized in Supplementary Data 1 . Telomere content of the controls anticorrelated with age ( r = −0.36, Spearman correlation; Supplementary Fig. 1a ). However, this age effect only has a low contribution to the strong correlation between the telomere content of the tumor and control samples ( r = 0.47 and r partial = 0.46 given the patient age, Spearman correlation, Supplementary Fig. 1b ). Thus, the association of tumor and control telomere content must mainly be caused by other genetic [27] , [28] , environmental [29] , or technical factors [26] . We normalized for these contributions by computing the ratio of tumor and control telomere content per individual. Most tumor samples had a lower telomere content than the matched control (Fig. 1a ). However, there were systematic differences between the different tumor types. Among those with the highest telomere content increase were osteosarcomas and leiomyosarcomas (median telomere content tumor/control log2 ratios = 0.7 and 0.6, respectively). A particularly low telomere content was found in colorectal adenocarcinoma and medulloblastoma (median telomere content tumor/control log2 ratios = −1.0). Fig. 1: Telomere content is increased in ATRX/DAXX trunc samples. a Overview of the telomere content distribution of all analyzed tumor types. The number of samples in each tumor type is indicated. Cohorts with sample sizes <15 are not shown. b TMM-associated mutations in different tumor types. c Telomere content in samples with different TMM-associated mutations. d TERT expression in samples with different TMM-associated mutations. The center lines of the boxplots are the medians, the bounds of the boxes represent the first and third quartiles, the upper and lower whiskers extend from the hinge to the largest or smallest value, respectively, no further than 1.5 × IQR from the hinge (where IQR is the interquartile range, or distance between the first and third quartiles). **** p < 0.0001, Wilcoxon rank-sum tests. Full size image Prevalence of TMM-associated mutations Different types of mutations in ATRX or DAXX , and at the TERT locus have been associated with ALT and telomerase activation, respectively. We therefore searched for these types of somatic mutations to infer the active TMM in a given tumor. Somatic mutations in ATRX , DAXX , or TERT were found in 16% of tumor samples. In total, 64 tumor samples had truncating ATRX ( n = 53) or DAXX alterations ( n = 11), and are referred to as ATRX/DAXX trunc in the following analysis. Of note, 10 of the 11 DAXX alterations were found in pancreatic endocrine tumors, while ATRX mutations were seen in a wider variety of entities. An additional 46 samples had nontruncating ATRX/DAXX simple nucleotide variants. TERT alterations (TERT mod ) were detected in 270 of the 2519 tumor samples (11%). The latter group comprised 198 activating C228T or C250T promoter mutations (of which 132 were obtained from the PCAWG simple nucleotide variant consensus calls and the remaining were detected with a targeted approach), 11 amplifications leading to at least six additional TERT copies, 55 structural variations within 20 kb upstream of TERT (TERTp SV ), and 6 samples with more than one of these modifications. Additionally, 18 tumor samples had both ATRX/DAXX truncating or other missense mutations and TERT alterations. “Enhancer hijacking” near the TERT transcription start site (TSS) has been described in neuroblastoma [8] and has recently been indicated in further cancer types [26] . In our data set, the strikingly focal distribution of structural variations upstream of the TERT TSS also points to this phenomenon (Supplementary Fig. 2 ). Further evidence is given by the direct overlap of 40% ( n = 25/62) of the juxtaposed positions within 20 kb upstream of the TERT TSS with enhancers from the dbSUPER database [30] . In contrast, only 13% ( n = 9/69) of the juxtaposed positions between 20 and 1000 kb corresponded to a predicted super-enhancer. Besides in melanoma (13% prevalence), chromophobe renal cell (9%), hepatocellular (9%), bladder transitional cell (4%), biliary (3%), and renal clear cell carcinoma (3%), previously undescribed TERTp SV in osteosarcoma (9%) and stomach adenocarcinoma (1%) were found. Moreover, the subtype-specific histological classification available in this study showed that TERTp SV were more frequent in liposarcoma (32%) than in leiomyosarcoma (7%). The tumor types with the highest prevalence of ATRX/DAXX trunc mutations were liposarcomas (32%), adult lower grade gliomas (28%), pancreatic endocrine tumors (23%), and osteosarcoma (17%; Fig. 1b and Supplementary Fig. 3a, b ), all of which have previously been associated with ALT [12] , [31] . TERT mod were most prevalent in transitional cell bladder cancer (70%), glioblastoma (67%), lower grade gliomas (61%), and melanoma (51%). The telomere content in TERT mod samples differed significantly from that in ATRX/DAXX trunc samples ( p = 1.1 × 10 −9 , Wilcoxon rank-sum test; Fig. 1c , a detailed overview is shown in Supplementary Fig. 4a ). On average, telomere content was gained in ATRX/DAXX trunc (mean telomere content tumor/control log2 ratio = 0.3), while telomere sequences were lost in TERT mod samples (mean telomere content tumor/control log2 ratio = −0.4). Samples with nontruncating ATRX/DAXX simple nucleotide variants had a similar telomere content as TERT mod samples ( p > 0.05, Wilcoxon rank-sum test), suggesting that most of the nontruncating ATRX/DAXX mutations are passenger events. In TERT mod samples and samples with unknown TMM, the telomere content correlated with TERT expression ( r = 0.20, Pearson correlation; p = 4.1 × 10 −10 , significance of fitted linear regression model) and TERT expression was significantly higher in TERT mod samples than in ATRX/DAXX trunc samples ( p = 1.3 × 10 −9 , Wilcoxon rank-sum test; Fig. 1d , detailed overviews are shown in Supplementary Figs. 3c and 4b ). High amount of telomere insertions in ATRX/DAXX trunc tumors To find insertions of telomeres into nontelomeric regions of the genome, we searched for tumor-specific discordant paired-end reads, where one end maps to the chromosome and the other end is telomeric. Exact positions of the insertions were determined from reads spanning the junction site and visual inspection (Fig. 2 ). Fig. 2: Examples of telomere insertions. a One-sided telomere insertion in liposarcoma sample SP121774. Blue tracks show the sequencing coverage; light blue represents clipped sequences. Individual reads are grey and clipped bases are colored. Dark grey reads represent the nontelomeric end of a discordant read pair. b Two-sided telomere insertion in breast adenocarcinoma sample SP5636. Nontelomeric clipped bases are transparent. c One-sided telomere insertion accompanied by copy number loss of the adjacent chromosome end in glioblastoma sample SP29559. Arches represent structural variations. d Multiple telomere insertions in a chromosome that underwent chromothripsis in melanoma sample SP124441. e One-sided telomere insertion accompanied by a translocation of the adjacent chromosome segment in pancreatic adenocarcinoma sample SP125764. Full size image Overall, 2683 telomere insertions were detected. These were distributed unevenly between samples and different tumor types (Fig. 3a ). Telomere insertions were found in 27% of the tumor samples, with counts ranging between 1 and 228 telomere insertion events. The tumor types with the highest amount of telomere insertions per tumor sample were liposarcoma, leiomyosarcoma, and osteosarcoma, all of which also had a relatively high mean telomere content. In fact, the number of telomere insertions positively correlated with the telomere content ( r = 0.19, Spearman correlation). Moreover, the number of telomere insertions was associated with the number of genomic breakpoints in the sample ( r = 0.38, Spearman correlation). To test for a synergistic effect, linear models that predict telomere insertions from telomere content and breakpoint abundance with and without an interaction term were computed. The models with the interaction term ( p = 8.8 × 10 −234 ) performed substantially better than purely additive models ( p = 5.8 × 10 −90 ). Fig. 3: Insertion of telomere sequences into nontelomeric chromosomal regions. a Number of telomere insertions in samples of different tumor types. The tumor types are sorted by mean telomere content tumor/control log2 ratios. Cohorts with sample sizes <15 are not shown. b Number of telomere insertions in samples with different TMM-associated mutations. c Number of breakpoints in samples with different TMM-associated mutations. d Percent of breakpoints coinciding with telomere insertions in samples with different TMM-associated mutations. The center line of the boxplot is the median, the bounds of the box represent the first and third quartiles, the upper and lower whiskers extend from the hinge to the largest or smallest value, respectively, no further than 1.5 × IQR from the hinge (where IQR is the interquartile range, or distance between the first and third quartiles). **** p < 0.0001, Wilcoxon rank-sum test. e Copy number changes of adjacent segments accompanying telomere insertions. “Complex” means that the copy numbers between segments differ in more than four copies. Overlaps with regions of chromothripsis are indicated. For telomere insertions that did not overlap with regions of chromothripsis, structural variations, or additional telomere insertions within 10 kb are indicated. Full size image There was clearly a higher percentage of samples with telomere insertions in ATRX/DAXX trunc tumors (80%) than TERT mod tumors (28%; Fig. 3b ). As expected, ATRX/DAXX trunc samples also had a higher number of breakpoints (mean = 733) than TERT mod samples (mean = 291; Fig. 3c ). Overall, the fraction of genomic breakpoints overlapping with telomere insertion sites was significantly higher in ATRX/DAXX trunc than TERT mod samples ( p = 1.7 × 10 −20 , Wilcoxon rank-sum test; Fig. 3d ). In agreement with the high breakpoint frequency, chromothripsis (numerous chromosomal rearrangements occurring in a single event) [32] was more prevalent in the ATRX/DAXX trunc samples (59%) compared to TERT mod samples (34%) and samples without ATRX/DAXX trunc and TERT mod mutations (29%). Similarly, ATRX/DAXX trunc samples were more likely to have an autosomal breakage-fusion-bridge (BFB) event (44%) than the remaining samples (TERT mod : 31%, other: 32%). In ATRX/DAXX trunc samples, autosomal chromosome arms that showed evidence for BFB cycles and chromothripsis had the highest incidence of telomere insertions (Supplementary Fig. 5 ). Correlation analysis of telomere insertions and mutations in telomere maintenance-associated genes from the TelNet database [33] [ http://www.cancertelsys.org/telnet ] revealed significant association with TP53 ( q = 1.9 × 10 −42 ), ATRX ( q = 2.6 × 10 −6 ), PLCB2 ( q = 7.8 × 10 −4 ), MEN1 ( q = 0.017), TSSC4 ( q = 0.017), RB1 ( q = 0.018), DAXX ( q = 0.019), and ABCC8 mutations ( q = 0.04, Wilcoxon rank-sum tests after Benjamini–Hochberg correction). 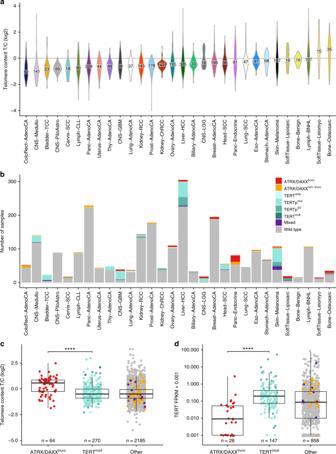Fig. 1: Telomere content is increased in ATRX/DAXXtruncsamples. aOverview of the telomere content distribution of all analyzed tumor types. The number of samples in each tumor type is indicated. Cohorts with sample sizes <15 are not shown.bTMM-associated mutations in different tumor types.cTelomere content in samples with different TMM-associated mutations.dTERTexpression in samples with different TMM-associated mutations. The center lines of the boxplots are the medians, the bounds of the boxes represent the first and third quartiles, the upper and lower whiskers extend from the hinge to the largest or smallest value, respectively, no further than 1.5 × IQR from the hinge (where IQR is the interquartile range, or distance between the first and third quartiles). ****p< 0.0001, Wilcoxon rank-sum tests. Most of these genes have been implicated in the maintenance of telomere length or structure in humans (Supplementary Table 1 ). The exceptions are PLCB2 and ABCC8 , whose homologues have so far only been reported in association with telomere length regulation in yeast [34] , [35] . The detected telomere insertions were scattered across different chromosomes and regions within the chromosome (Supplementary Fig. 6 ). No clear preferential insertion sites were identified, but several de novo telomere junctions occurred at the chromosome ends (5% within 50 kb of the first or last chromosomal segment). A total of 44% of the telomere insertions were in genes, and 8% of these disrupted exons. Several tumor suppressor genes were affected, e.g., CHEK1 encoding for a protein involved in cell cycle arrest upon DNA damage [36] (Fig. 2a ). Of note, patterns of microhomology were observed in 79% of telomere insertions with t-type repeats at the junction site (Supplementary Fig. 7 ). Frequent copy number losses at telomere insertion sites Most of the telomere insertions were one-sided (98%), i.e., telomere sequences were only attached to one side of the breakpoint (Fig. 2a ). Telomere insertions were defined as two-sided, if there was a second telomere insertion event downstream in the opposite orientation (Fig. 2b ). Two-sided telomere insertions can occur via a telomere sequence that bridges two chromosome fragments or, alternatively, telomere sequences are independently fused to both ends of the chromosome break. Reads supporting the first scenario were found in 14 of the 25 two-sided telomere insertions pairings. For the other cases, the inserted repeat sequence was too long to distinguish between the two scenarios. Because so many breakpoints were one-sided, we investigated the fate of the corresponding broken fragment using complementary information from copy number changes and structural variation annotation (Fig. 3e ). As expected, one-sided telomere insertions coincided most frequently with copy number loss of the adjacent segment (46%, Fig. 2c ). In contrast, copy number gains of the fragment were rare (6%). Surprisingly, telomere insertions were frequently located at copy-number neutral sites (42%). Overlaps with regions of chromothripsis were found for 25% and structural variations without chromothripsis overlap (including telomere insertions) were detected near the insertion site for 28% of the copy-number neutral cases (Fig. 2d, e ). The remaining telomere insertions at copy-number neutral sites are likely to be subclonal (Supplementary Fig. 8a ) or have undetected structural variations nearby (Supplementary Fig. 8b ). Occasional TERRA expression at telomere insertions ALT-positive tumors have been associated with elevated levels of long noncoding telomeric repeat-containing RNA (TERRA) [16] . We searched for TERRA expression in the RNA-sequencing data of 867 tumor samples. In line with the results of Barthel et al. [26] , TERRA levels were higher in ATRX/DAXX trunc compared to TERT mod samples ( p = 5.0 × 10 −7 , Wilcoxon rank-sum test, Supplementary Fig. 9 ). In 16 samples, evidence for TERRA expression at telomere insertion sites was found. For most of these, the number of split reads supporting TERRA expression was low (between 1 and 8 reads). However, 146 TERRA reads expressed from only two telomere insertion sites were detected in an ATRX/DAXX trunc liposarcoma sample, making up almost 6% of its total TERRA read count. This percentage is likely to be notably higher, as the short read length does not allow assignment of the total number of TERRA reads stemming from these telomere insertions. Thus, TERRA is not exclusively transcribed from TSSs in the subtelomeric region but can also arise from telomere insertions. Of note, these telomere insertion transcripts do not always contain the canonical UUAGGG repeat but can also be composed of the reverse complement CCCUAA. Enrichment of singleton TVRs in ATRX/DAXX trunc samples It has previously been shown that ALT leads to an increased integration of TVRs into telomeres, the most common ones being hexamers of the type NNNGGG [15] . To detect differences in the telomere composition of ATRX/DAXX trunc and TERT mod tumors, we therefore searched for NNNGGG repeats in telomere reads. The most frequent TVRs across all tumor samples were TGAGGG, TCAGGG, and TTGGGG (Supplementary Fig. 10 ), which are known to be enriched in proximal telomeric regions [2] , [3] . These and the seven other most frequent TVRs (TAAGGG, GTAGGG, CATGGG, TTCGGG, CTAGGG, TTTGGG, and ATAGGG) were chosen to search for common telomere repeat combinations. For this, the neighboring 18 base pairs on either side of the TVRs were determined (Supplementary Data 2 ). Most TVRs were surrounded by many different pattern combinations (e.g., TTGGGG). Others were dominated by a certain repeat context, which was similar in ATRX/DAXX trunc and TERT mod tumors (e.g., CATGGG or ATAGGG). However, TTCGGG stood out, as 41% of the TVRs in ATRX/DAXX trunc samples were surrounded by canonical t-type repeats, whereas this context was observed for only 4% of TTCGGG TVRs in TERT mod tumors. Following up on this observation, we compared variant hexamers surrounded by at least three t-type repeats on either side (“singletons”) to TVRs in an arbitrary sequence context. This revealed that singletons are generally well suited to distinguish ATRX/DAXX trunc from TERT mod samples (Fig. 4a , an overview of all patterns is shown in Supplementary Fig. 11 ). The remaining variant analysis therefore focused on such TVR singletons. CATGGG was excluded as it did not occur as singletons. For the other TVRs, the median of absolute counts varied between 12 and 100, but counts in individual tumor samples reached >10,000 (Supplementary Fig. 12 ). Fig. 4: Singleton TVRs enriched or depleted in ATRX/DAXX trunc samples. a Receiver operating characteristic for the classification of samples with ALT-associated mutations from telomere variant repeats. Red: no specific sequence context required. Blue: singletons ((TTAGGG) 3 -NNNGGG-(TTAGGG) 3 ). The more the area under the curve (AUC) deviates from 0.5, the better the repeat occurrence distinguishes ATRX/DAXX trunc from TERT mod samples. b Pattern count tumor/control log2 ratios of all patients plotted against telomere content tumor/control log2 ratios for selected singletons. The regression line through the TERT mod samples is shown in green and is defined as the expected pattern count in the following. c Distance to the expected singleton repeat count in ATRX/DAXX trunc and TERT mod samples. The center line of the boxplot is the median, the bounds of the box represent the first and third quartiles, the upper and lower whiskers extend from the hinge to the largest or smallest value, respectively, no further than 1.5 × IQR from the hinge (where IQR is the interquartile range, or distance between the first and third quartiles). **** p < 0.0001; *** p < 0.001, Wilcoxon rank-sum tests after Bonferroni correction. The profiles of all analyzed patterns are shown in Supplementary Figs. 11 and 13 . Full size image As expected, normalized singleton repeat counts generally rose with increasing telomere content (Fig. 4b , an overview of all patterns is shown in Supplementary Fig. 13 ). However, TGAGGG, TCAGGG, TTGGGG, and TTCGGG singletons had significantly higher counts than expected in ATRX/DAXX trunc compared to TERT mod samples ( p = 7.3 × 10 −11 , 7.9 × 10 −6 , 5.6 × 10 −4 , and 5.8 × 10 −13 , respectively, Wilcoxon rank-sum test after Bonferroni correction; Fig. 4c ). Especially, TGAGGG and TTCGGG seemed to be highly interspersed in a subset of ATRX/DAXX trunc tumors. In contrast, TTTGGG singletons were observed less frequently in ATRX/DAXX trunc tumors ( p = 3.8 × 10 −12 , Wilcoxon rank-sum test after Bonferroni correction). 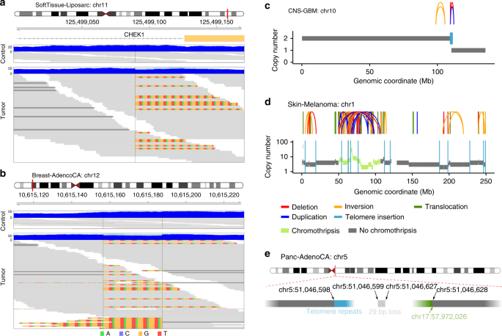Fig. 2: Examples of telomere insertions. aOne-sided telomere insertion in liposarcoma sample SP121774. Blue tracks show the sequencing coverage; light blue represents clipped sequences. Individual reads are grey and clipped bases are colored. Dark grey reads represent the nontelomeric end of a discordant read pair.bTwo-sided telomere insertion in breast adenocarcinoma sample SP5636. Nontelomeric clipped bases are transparent.cOne-sided telomere insertion accompanied by copy number loss of the adjacent chromosome end in glioblastoma sample SP29559. Arches represent structural variations.dMultiple telomere insertions in a chromosome that underwent chromothripsis in melanoma sample SP124441.eOne-sided telomere insertion accompanied by a translocation of the adjacent chromosome segment in pancreatic adenocarcinoma sample SP125764. This seemingly ALT-specific TVR enrichment or depletion occurred in different tumor types, with the highest prevalence in leiomyosarcomas (60%), pancreatic endocrine tumors (42%), liposarcomas (37%), osteosarcomas (29%), and lower grade gliomas (28%; Supplementary Table 2 ). In the ATRX/DAXX trunc samples, singleton TVR occurrences correlated with each other (Supplementary Fig. 14 ). The strongest correlations were between TGAGGG occurrence and TTCGGG and TTGGGG singletons ( r = 0.57 and r = 0.58, respectively, Spearman correlation). ALT prediction ALT has several different hallmarks with which it can be reliably identified [11] . However, most of these are not detectable in short-read WGS data. Using ATRX/DAXX trunc as indicators of ALT, we have shown several possible TMM classification features based on WGS. Most ATRX/DAXX trunc samples are already separated well from TERT mod samples by nonsupervised clustering of normalized TGAGGG, TCAGGG, TTGGGG, TTCGGG, and TTTGGG singleton repeat counts (Supplementary Fig. 15 ). As expected, the clusters of ATRX/DAXX trunc samples had a high telomere content and a high number of telomere insertions relative to the total number of breakpoints. These features were further used to build a random forest classifier distinguishing ATRX/DAXX trunc from TERT mod samples (area under the curve: 0.95; sensitivity: 0.73; specificity: 0.99; all after 10-fold cross-validation). 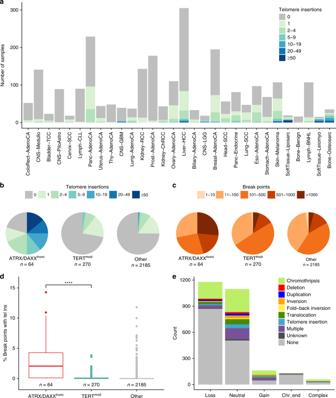Fig. 3: Insertion of telomere sequences into nontelomeric chromosomal regions. aNumber of telomere insertions in samples of different tumor types. The tumor types are sorted by mean telomere content tumor/control log2 ratios. Cohorts with sample sizes <15 are not shown.bNumber of telomere insertions in samples with different TMM-associated mutations.cNumber of breakpoints in samples with different TMM-associated mutations.dPercent of breakpoints coinciding with telomere insertions in samples with different TMM-associated mutations. The center line of the boxplot is the median, the bounds of the box represent the first and third quartiles, the upper and lower whiskers extend from the hinge to the largest or smallest value, respectively, no further than 1.5 × IQR from the hinge (where IQR is the interquartile range, or distance between the first and third quartiles). ****p< 0.0001, Wilcoxon rank-sum test.eCopy number changes of adjacent segments accompanying telomere insertions. “Complex” means that the copy numbers between segments differ in more than four copies. Overlaps with regions of chromothripsis are indicated. For telomere insertions that did not overlap with regions of chromothripsis, structural variations, or additional telomere insertions within 10 kb are indicated. The variables with the highest importance for the classification were the divergence of observed TTTGGG and TTCGGG singleton TVRs from the expected count, the number of breakpoints and the number of telomere insertions (Supplementary Table 3 ). It may be pivotal for further understanding of this mechanism to determine the causal relationship between these features and the ALT phenotype. The scores resulting from the classifier can be interpreted as an ALT probability. As expected, ATRX/DAXX trunc had a high ALT probability (mean = 0.91), while TERT mod samples had a low ALT probability (mean = 0.13, Supplementary Fig. 16 ). A total of 17 samples without ATRX/DAXX trunc mutations had an ALT probability of over 0.9, of which three had nontruncating ATRX/DAXX mutations and one sample had a frameshift insertion in ATRX and a TERT amplification (11 TERT copies, triploid). Across the entire dataset, most samples had a low ALT probability (Supplementary Fig. 17 ), suggesting that their TMM is telomerase based. This included some samples with ATRX/DAXX missense mutations, suggesting that the mutations in those samples may be more of a passenger event than functionally relevant. Tumor types with a high ALT probability were leiomyosarcoma, osteosarcoma, pancreatic endocrine tumors, and liposarcomas, in keeping with the known high prevalence of ALT in these entities [37] , [38] , [39] . In this study, we have shown that the presence of ALT-associated mutations in tumors correlates with increased telomere content, enrichment of isolated TVRs in t-type context (singletons), a higher number of genomic breakpoints, and intrachromosomal telomere insertions (Fig. 5 ). In contrast, tumors with mutations associated with a possible telomerase activation showed moderate decrease of telomere content and increased TERT expression. Hence, TERT reactivation may not suffice to fully counteract the telomere loss associated with high proliferation and/or occur when advanced telomere attrition increases the selective pressure to activate telomere maintenance. The observed telomere content increase in ATRX/DAXX trunc versus the decrease in TERT mod samples is in agreement with the recent findings of Barthel et al. [26] . The higher telomere content in ATRX/DAXX trunc tumors indicates that the negative feedback loop that constrains telomere elongation to a physiological level in healthy telomerase-expressing cells [40] , [41] is bypassed by the ALT process, while it seems to remain intact in telomerase-positive tumors. In addition to telomere elongation, the increase of telomere content in ALT-positive tumors detected by sequencing-based methods may partly stem from aberrant intrachromosomal telomere insertions [18] or extrachromosomal telomeric DNA [42] . Although almost all tumors must maintain their telomeres [43] , we only detected somatic mutations highly associated with ALT or telomerase activation in a subset of the samples. In tumors arising from tissues with high rates of self-renewal, telomerase is likely to already be epigenetically activated in the cell of origin [44] , [45] . Thus, telomere maintenance activating mutations occur more frequently in tumors derived from slowly replicating cells [46] . In line with this assumption, we observed high rates of TMM-associated mutations in brain, liver, bladder, and kidney tumors and TERT expression despite lack of TMM-associated mutations in lymphomas, tumors of the gastrointestinal tract, and female reproductive system. The exceptions were pilocytic astrocytoma, pancreatic, and prostate adenocarcinoma, which all originate from slowly replicating tissues, but had almost no TMM-associated alterations. In pancreatic and prostate cancer, TERT activity has been detected [47] , [48] , suggesting other means of telomerase activation. In pilocytic astrocytoma, neither telomerase expression/activity nor ALT was observed, but preALT characteristics have been reported [49] , [50] . Therefore, a TMM may only be fully activated upon progression of this slow-growing tumor type. Medulloblastoma samples only had a TERT mod frequency of 14% and one of the lowest average telomere contents in our study. While TERTp mut tend to occur in older patients of the SHH subgroup, the TERT promoter is frequently methylated in younger SHH patients and other medulloblastoma subgroups [51] . Interestingly, SHH medulloblastomas are thought to arise from granule neuron precursor cells [52] . This is a cell type with an extremely high rate of turnover during development and infancy, which may explain the TERT promoter methylation in younger SHH patients. In agreement with data suggesting that TERT expression is higher in TERTp mut than in TERT promoter methylated medulloblastomas [51] , we found that the telomere content was significantly higher in medulloblastomas with TERT mod than in those without ( p = 0.0045, Wilcoxon rank-sum test). Fig. 5: Genomic footprints of telomerase-mediated telomere elongation and ALT. It is known that telomeres elongated by telomerase have a homologous length with few TVRs in distal telomeric regions (left), while ALT telomeres have heterogeneous lengths with an increased amount of TVRs (right). Moreover, ALT cells have abundant extrachromosomal telomeric sequences. From this study, we conclude that the chromosomes of ALT cells have a higher number of aberrant interstitial telomere insertions, most of which are one-sided and accompanied by a loss of the adjacent chromosomal segment. We also showed that several TVRs occurring as singletons are more abundant in ALT telomeres, while one singleton (TTTGGG) was more abundant in telomerase-elongated telomeres. Please note that it is currently undetermined whether the different types of singletons are located in proximal or distal telomeric regions. Full size image In our study, we systematically mapped telomere insertions into nontelomeric genomic regions using WGS data. They were most frequently accompanied by a loss of the adjacent chromosomal segment or located at copy-number neutral sites. Surprisingly, the latter telomere insertions were rarely two-sided and chromothripsis or other structural variations in the adjacent genomic regions occurred only in about half of the cases. As broken chromosome ends are highly unstable, the remaining segments must have undetected structural rearrangements, such as subclonal copy number changes or undetected DNA fusions. Taken together, the results suggest that we observe telomere healing or capture [20] , [21] rather than telomere insertions followed by chromosomal instabilities [18] , [53] . As microhomology around telomere insertion sites was frequent, the sequences were probably inserted by nonhomologous end-joining [54] or a microhomology-mediated mechanism [55] . Telomere insertions were particularly frequent in ATRX/DAXX trunc tumors, in which the abundant extrachromosomal telomeric DNA expands the telomere template pool for microhomology-mediated double-strand repair. We speculate that in this cellular environment, a high load of genomic breakpoints subsequently leads to the observed disproportionately increased number of telomere capture-like events. Due to the stochastic nature of ALT, the likelihood of telomere crisis is elevated, an event that can induce BFB cycles [56] , [57] and chromothripsis [58] . Nevertheless, ALT can also stabilize telomeres, which has been shown to counteract genomic instability in certain instances [59] . Either scenario may account for the higher prevalence of chromothripsis and BFB events in ATRX/DAXX trunc cases observed in this study. Together with the correlation of telomere insertions and mutations in TP53 , RB1 , MEN1 , ATRX , and DAXX , these findings suggest that genome instability and the ALT phenotype are prerequisites for a high number of telomere insertions. Mutations in TP53 , RB1 , and MEN1 have been associated with impaired DNA damage response and repair [60] , [61] , [62] . This may make telomere crisis and genomic rearrangements more likely, while at the same time preventing apoptosis or senescence. Supporting all of these associations, an increased incidence of ALT in combination with chromothripsis was observed in SHH medulloblastomas with TP53 germline or somatic mutations [59] . Telomere elongation by ALT or telomerase enriches distinct TVRs [15] . Here, we report a stronger association of singleton TVRs with ATRX/DAXX trunc mutations than TVRs in an arbitrary context. The increase of TVRs has been attributed to the inclusion of subtelomeric regions during ALT via homologous recombination [14] . Whether telomeric sequences with lower TVR density are under positive selection or regions with higher TVR density are under negative selection remains to be clarified. A possible function for TVRs has been reported in ALT-positive cell lines, where TCAGGG repeats that recruit nuclear receptors were enriched [14] , [18] . This enrichment was confirmed in a subset of primary ATRX/DAXX trunc tumor samples in our study. However, we found a more pronounced enrichment of TTCGGG or TGAGGG. While TGAGGG has previously been associated with ALT [14] , the high prevalence of TTCGGG singletons in ALT is a novel discovery. No proteins with strong affinity to these two TVRs are currently known. This may indicate a more passive mode of action, for instance deprotection of telomeres by shelterin displacement [14] , and/or alteration of the telomeric G-quadruplex conformation [15] . Notably, we report for the first time that TTTGGG singletons but not TTTGGG in arbitrary context were depleted in ATRX/DAXX trunc samples. This finding underlines the necessity to consider the sequence context of TVRs. None of the current models of ALT provide an explanation for this specific TVR depletion. The methodologies presented here expand the established telomere content estimation from genomic sequencing by the context-dependent analysis of TVRs and telomere insertions. By applying them within a large-scale pan-cancer study, we provide a valuable resource for the further characterization of different TMMs in cancer cells based on WGS data. Sequencing data WGS and expression data were obtained from the ICGC/TCGA PCAWG project [23] . The WGS reads of tumor and control samples were aligned with bwa-mem by the PCAWG-tech group. Control samples were usually blood. In a small number of cases, the controls were obtained from tumor-adjacent or other tissue [23] . Tumors with multiple samples were excluded from this study, as well as one sample pair with reads shorter than 30 bp. Expression data was in the format of normalized RNA read counts per gene and only available for 1033 of 2519 patients. RNA sequencing BAM files aligned with STAR by the PCAWG-tech group were available for 867 tumor samples. To avoid confusion, we used the name “(central nervous system) CNS-LGG” (lower grade glioma, i.e., grades II and III) for the “CNS-Oligo” tumor type, because several samples in this cohort did not have the genetic markers (i.e., 1p/19q co-deletions) for oligodendroglioma required by the WHO [63] . 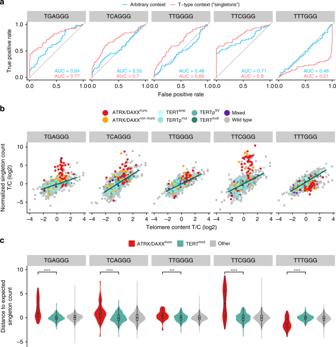Fig. 4: Singleton TVRs enriched or depleted in ATRX/DAXXtruncsamples. aReceiver operating characteristic for the classification of samples with ALT-associated mutations from telomere variant repeats. Red: no specific sequence context required. Blue: singletons ((TTAGGG)3-NNNGGG-(TTAGGG)3). The more the area under the curve (AUC) deviates from 0.5, the better the repeat occurrence distinguishes ATRX/DAXXtruncfrom TERTmodsamples.bPattern count tumor/control log2 ratios of all patients plotted against telomere content tumor/control log2 ratios for selected singletons. The regression line through the TERTmodsamples is shown in green and is defined as the expected pattern count in the following.cDistance to the expected singleton repeat count in ATRX/DAXXtruncand TERTmodsamples. The center line of the boxplot is the median, the bounds of the box represent the first and third quartiles, the upper and lower whiskers extend from the hinge to the largest or smallest value, respectively, no further than 1.5 × IQR from the hinge (where IQR is the interquartile range, or distance between the first and third quartiles). ****p< 0.0001; ***p< 0.001, Wilcoxon rank-sum tests after Bonferroni correction. The profiles of all analyzed patterns are shown in Supplementary Figs.11and13. 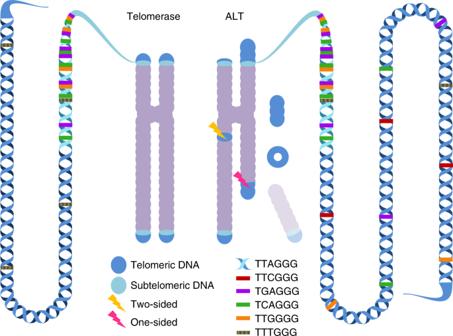Fig. 5: Genomic footprints of telomerase-mediated telomere elongation and ALT. It is known that telomeres elongated by telomerase have a homologous length with few TVRs in distal telomeric regions (left), while ALT telomeres have heterogeneous lengths with an increased amount of TVRs (right). Moreover, ALT cells have abundant extrachromosomal telomeric sequences. From this study, we conclude that the chromosomes of ALT cells have a higher number of aberrant interstitial telomere insertions, most of which are one-sided and accompanied by a loss of the adjacent chromosomal segment. We also showed that several TVRs occurring as singletons are more abundant in ALT telomeres, while one singleton (TTTGGG) was more abundant in telomerase-elongated telomeres. Please note that it is currently undetermined whether the different types of singletons are located in proximal or distal telomeric regions. A detailed overview of tumor type abbreviations with the included subtypes is given in Supplementary Table 4 . Mutation data Somatic simple nucleotide, structural variations, and copy numbers were obtained from the PCAWG consensus calls (Synapse IDs syn7364923, syn7596712, and syn8042992, respectively). Structural variations were not available for 24 tumor samples. Telomere read extraction and computational telomere content estimation The telomere content of WGS samples was determined using the software tool TelomereHunter [64] . In short, telomeric reads containing six nonconsecutive instances of the four most common telomeric repeat types (TTAGGG, TCAGGG, TGAGGG, and TTGGGG) were extracted. For the further analysis, only unmapped reads or reads with a very low alignment confidence (mapping quality lower than 8) were considered. The telomere content was determined by normalizing the telomere read count by all reads in the sample with a GC content of 48–52%. Determining TMM-associated mutations Samples with a truncating ATRX or DAXX alteration (frame-shift insertion/deletion, stop-codon gain, or structural variation breakpoint within the gene) were defined as ATRX/DAXX trunc , samples with other simple nucleotide variants were defined as ATRX/DAXX non-trunc . Deletions that only affected intronic regions of ATRX were not considered. Of note, a frame-shift deletion called in the tumor sample of donor SP112201 was excluded as a false positive after visual inspection in the Integrative Genomics Viewer (IGV) [65] , [66] . Samples with a structural variation breakpoint on the plus strand 20 kb upstream of TERT the TSS were defined as TERTp SV . TERT amp samples had at least six additional copies of the TERT gene compared to the mean ploidy of the sample. Tumor samples with a C228T or C250T TERT promoter mutation were defined as TERTp mut . Due to the low sequencing coverage at the TERT promoter, these mutations were called using less stringent criteria (at least two reads with the mutated base, mutational frequency of at least 20%) in addition to the PCAWG consensus single nucleotide variant (SNV) calls (Synapse ID syn7364923). If multiple of these TERT modifications were present, the sample was defined as TERT mult . Samples with these TERT alterations were summarized as TERT mod . Samples without any of these alterations were defined as “wild type”. If a sample had both a TERT mod alteration and an ATRX/DAXX alteration, it was defined as “mixed”. For some analyses, ATRX/DAXX non-trunc , mixed and wild-type samples were summarized as “other”. Overlap of juxtaposed positions upstream of TERT and predicted super-enhancers For the closest structural variation (SV) of each tumor sample to the TERT TSS, the juxtaposed genomic coordinates were compared to 65,950 predicted super-enhancers from the dbSUPER database [30] . Only SVs on the plus strand and within 1 mb of the TERT TSS were considered. Overlaps of juxtaposed positions with super-enhancer sites were defined as direct overlaps. Super-enhancer sites within 1 mb of the juxtaposed position were defined as indirect overlaps. Telomere insertion detection To find insertions of telomeric sequences into nontelomeric regions in the genome, we searched for tumor-specific discordant paired-end reads, where one end was an extracted telomere read and the other end was nontelomeric and uniquely mapped to a chromosome (mapping quality > 30). In 1 kb regions containing at least three discordant reads in the tumor sample and none in the matching control, exact positions of telomere insertions were defined by at least three split reads spanning the insertion site. The split reads had to contain at least one TTAGGG repeat. Regions with discordant read pairs in at least 15 control samples were excluded. Finally, the insertion sites were visualized using IGV [65] , [66] to identify and remove remaining false positives. A telomere insertion was defined as two-sided if another telomere insertion in opposite orientation was found in the downstream 10 kb of the reference genome with the same repeat on the forward strand. Otherwise it was defined as one-sided. Breakpoint detection Breakpoints were obtained from the consensus breakpoint list of structural and copy number variation calls (Synapse ID syn8042992). In short, six copy number detection tools were run on all samples, including the consensus structural variations breakpoints. From the obtained chromosomal segments of the individual callers another set of consensus breakpoints was calculated. Chromothripsis detection To identify chromothripsis events, we extended the set of statistical criteria proposed by Korbel and Campbell [67] . The basic idea is to determine whether there is a statistically significant number of interleaved structural variants in a contiguous genomic region. We did this by constructing a graph whose nodes correspond to SVs and whose edges connect interleaved SVs. The identified clusters of SVs were also tested for the presence of alternating copy number and loss-of-heterozygosity patterns. The resulting chromothripsis calls were validated visually. The full description of the methodology and the detailed patterns of chromothripsis events in the genomes are described in a separate study [24] . Only high-confidence chromothripsis calls were included in this analysis. BFB detection At least two fold-back inversions on the same chromosome arm were defined as BFB events. Fold-back inversions had to fulfill the following requirements adapted from Cheng et al. [68] : (1) the two breakpoints of the inversion are less than 20 kb apart; (2) the inversion does not have a reciprocal partner, such that inversion1_start < inversion2_start < inversion1_end < inversion2_end; and (3) there is a copy number change at the inversion site. Copy number changes at telomere insertion sites Copy numbers of chromosomal segments were obtained from the PCAWG consensus calls (Synapse ID syn8042992). Copy numbers reveal gains or losses of chromosomal segments based on coverage and B-allele frequency, but were here limited to segments of at least 10 kb. The breakpoint estimations could differ from the actual site by up to 50 kb. Therefore, telomere insertions were assigned to the closest breakpoint within 50 kb. If there was no breakpoint within 50 kb or the copy numbers at either side of the telomere insertion were the same, the copy number change at the telomere insertion was defined as neutral. Structural variations near telomere insertion sites Structural variation annotation was obtained from the PCAWG consensus calls (Synapse ID syn7596712), which was based on discordant mate pairs and split reads, providing exact breakpoints. Because copy number variations smaller than 10 kb were not detected by copy number callers, small deletions next to the telomere insertion site may be missed. We therefore searched for structural variations within 10 kb of a telomere insertion to detect these cases. Candidate gene selection for correlation analysis A list of 1725 telomere maintenance associated human genes was obtained from TelNet [33] on February 20, 2017. After removing genes without a unique Ensembl IDs in the GENCODE [69] v19 HAVANA annotation, the remaining 1686 genes were used for correlation of telomere insertions and simple nucleotide variants. TERRA detection TelomereHunter was run on RNA-Seq BAM files to count reads containing at least k nonconsecutive instances of the four most common telomeric repeat types (TTAGGG, TCAGGG, TGAGGG, and TTGGGG). The repeat threshold k was chosen depending on the read length: k = 7 for 45–50 bp, k = 10 for 75–76 bp, and k = 14 for 99–101 bp. The resulting TERRA read counts were normalized by the total number of reads in the sample. For better readability, this number was multiplied by 1 Mio. Detection of TVRs TVRs were detected by searching for hexamers of the type NNNGGG in the extracted telomere reads. Each base was required to have a base quality of at least 20. The neighboring 18 bp on either side of the TVR were determined. For further analysis, NNNGGG TVRs were once computed for arbitrary context and once for t-type context ((TTAGGG) 3 -NNNGGG-(TTAGGG) 3 , also called “singletons”). The absolute counts were normalized to the total number of reads in the sample. The expected pattern counts in arbitrary context were calculated as: telomere content tumor/control log2 ratio. The expected singleton counts at different telomere content tumor/control log2 ratios were taken from the regression line through TERT mod samples. The singleton occurrence heatmap was generated using the R package ComplexHeatmap [70] . Classifier for predicting active TMMs A random forest classifier to distinguish ATRX/DAXX trunc and TERT mod samples was built using the R packages “randomForest” [71] and “caret” [72] with the following eight features: telomere content tumor/control log2 ratio, number of telomere insertions, number of breakpoints, and the distance of TGAGGG, TCAGGG, TTGGGG, TTCGGG, and TTTGGG singletons (i.e., repeats in a t-type context) to their expected occurrence. To deal with the imbalance in the data set (i.e., 266 TERT mod samples versus 63 ATRX/DAXX trunc samples without missing data), the model was trained with a down-sampled training set. The performance was determined using 10-fold cross-validation. Statistics Differences between ATRX/DAXX trunc and TERT mod samples in terms of telomere content, percent breakpoints with telomere insertions, and singleton repeat abundance were tested using two-sided Wilcoxon rank-sum tests. Singleton repeat abundance p -values were corrected for multiple testing using the Bonferroni method. To reduce the influence of outliers, correlation coefficients were calculated with the Spearman method. Correlation between control telomere content and age as well as tumor and control telomere content was tested with linear regression. All statistical analyses were carried out using R (R Foundation for Statistical Computing). Reporting summary Further information on research design is available in the Nature Research Reporting Summary linked to this article.